Comprehensive bioimaging with fluorinated nanoparticles using breathable liquids Fluorocarbons are lipophobic and non-polar molecules that exhibit remarkable biocompatibility, with applications in liquid ventilation and synthetic blood. The unique properties of these compounds have also enabled mass spectrometry imaging of tissues where the fluorocarbons act as a Teflon-like coating for nanostructured surfaces to assist in desorption/ionization. Here we report fluorinated gold nanoparticles (f-AuNPs) designed to facilitate nanostructure imaging mass spectrometry. Irradiation of f-AuNPs results in the release of the fluorocarbon ligands providing a driving force for analyte desorption. The f-AuNPs allow for the mass spectrometry analysis of both lipophilic and polar (central carbon) metabolites. An important property of AuNPs is that they also act as contrast agents for X-ray microtomography and electron microscopy, a feature we have exploited by infusing f-AuNPs into tissue via fluorocarbon liquids to facilitate multimodal (molecular and anatomical) imaging. Fluorocarbons have remarkable chemical and physical characteristics that allow unique surface properties, high stability, low reactivity and an ability to solubilize gases. The biocompatibility of fluorocarbons has been demonstrated [1] , [2] , [3] , [4] , [5] and has inspired researchers to utilize these compounds for a wide range of biomedical and research applications. For example, these properties have enabled fluorocarbons to be applied in areas as diverse as surface coatings [6] , drug delivery [4] , liquid ventilation [1] , synthetic blood [2] and several imaging modalities [4] , [5] , [7] , [8] including mass spectrometry imaging [9] . Mass spectrometry imaging facilitates the spatially resolved mass analysis of metabolites in situ [10] , [11] , [12] where investigators have a choice of multiple technologies each with their inherent advantages and disadvantages [9] , [13] , [14] , [15] , [16] , [17] , [18] . These techniques include matrix-assisted laser desorption/ionization mass spectrometry (MALDI-MS) [15] , secondary ion mass spectrometry [13] , desorption electrospray ionization [14] , MALDESI [18] , and others [9] , [16] , [17] , [19] . While there have been some successful developments in low energy [20] and low background [21] matrices for MALDI-MS, the most widely used of these technologies, these matrices do not facilitate multiple modes imaging. Gold nanoparticles (AuNPs) are well known as contrast agents for X-ray imaging technologies [22] , [23] , [24] and electron microscopy [25] . For example, the attenuation property of X-rays by AuNPs has led to their use as contrast agents in computed tomography (CT) imaging [26] , [27] . AuNP have also been exploited for mass spectrometry molecular imaging, thus presenting a single platform capable of supporting comprehensive bioimaging. However, AuNPs’ ability to facilitate molecular imaging via mass spectrometry is limited due to the required high laser energies, resulting in significant fragmentation and generally poor sensitivity [28] . While AuNPs are attractive biomedical imaging agents, they have not been explored as agents to correlate structure with molecular information given their limitations with mass spectrometry. Indeed, when performing mass spectrometry-based metabolomic imaging, correlating metabolite localization patterns with tissue anatomy is key to data interpretation but has represented a serious challenge. Traditionally, correlations have been based on immunohistochemistry. Given that immunohistochemistry chemically alters tissue sections immunohistochemistry and mass spectrometry imaging cannot be performed on the same tissue samples. Here we introduce f-AuNPs as an agent for nanostructure imaging mass spectrometry (NIMS). The use of fluorocarbons as a covalent modification of AuNPs for this application is a natural choice given the history [17] of fluorocarbons facilitating NIMS, specifically nanostructured silicon has benefited from fluorine modifications [9] . Fluorinated silicon nanostructures used for laser desorption/ionization have been shown to generate low background interference, have minimal ultraviolet absorbance, generate little fragmentation and, given their unique super-hydrophobicity, readily allow for the desorption of metabolites from their surface with high sensitivity. In addition, fluorous initiators containing amino groups can be used to promote [M−H] − production [29] , [30] , which, similar to basic MALDI matrices [31] , [32] , have been successfully applied to mass spectrometry imaging of central carbon metabolites. In addition to mass spectrometry imaging, f-AuNPs, unlike MALDI matricies, are also capable of acting as contrast agents for X-ray analysis and electron microscopy [22] , [23] , [24] , [25] . We demonstrate f-AuNP multimodal imaging to generate X-ray (μCT) and electron microscopy structural images, as well as facilitating mass spectrometry imaging, providing both anatomical and molecular information. Fluorinated AuNPs for mass spectrometry imaging Given the advantages that fluorocarbon modifications impart on silicon nanostructure mass spectrometry imaging, our goal in these studies was to adapt fluorocarbon ligands to the more versatile AuNPs. In laser desorption/ionization experiments, silicon nanostructures and AuNPs absorb energy extremely well in the ultraviolet region [33] , [34] , [35] and in the case of AuNPs, the core can reach ~2,000 K in a few nanoseconds [36] . While AuNPs alone have limited ability to facilitate molecular imaging via mass spectrometry due to the required high laser energies resulting in significant fragmentation and generally poor sensitivity [28] . AuNPs with fluorocarbon ligands (f-AuNPs) are designed to initiate the desorption/ionization mass spectrometry event while attenuating energy transfer to the analyte. This is accomplished through the fluorinated ligand, which serves to insulate the analyte from the thermal energy of the AuNP (~2,000 K) while the laser-induced release of the ligand allows it to act as a conduit for analyte desorption. We posit that the thermal desorption of the ligand provides enough kinetic energy to drive analyte desorption into the gas phase with minimal energy input, as illustrated in Fig. 1 . 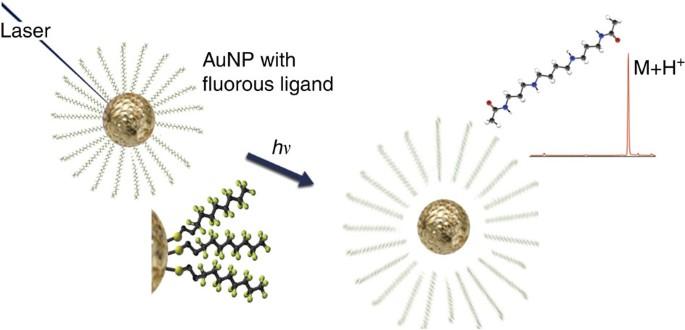Figure 1: Decoupling laser-induced nanoparticle heating from desorption/ionization. Schematic illustration of the possible desorption mechanism: on irradiation, gold core efficiently absorbs the laser energy and transfers the energy to thermally release fluorinated ligands. The desorbed fluorinated ligands provide the kinetic energy (and driving force) for analyte desorption and serve to protect the analyte from thermal degradation. Protonated diacetylspermine is shown as an example of f-AuNP desorption/ionization. Figure 1: Decoupling laser-induced nanoparticle heating from desorption/ionization. Schematic illustration of the possible desorption mechanism: on irradiation, gold core efficiently absorbs the laser energy and transfers the energy to thermally release fluorinated ligands. The desorbed fluorinated ligands provide the kinetic energy (and driving force) for analyte desorption and serve to protect the analyte from thermal degradation. Protonated diacetylspermine is shown as an example of f-AuNP desorption/ionization. Full size image In a representative experiment, we have demonstrated the utility of these f-AuNPs to carry out MS analysis of pure standards ( Supplementary Fig. 1 ) and human plasma ( Supplementary Fig. 2 ) using two instruments designed for MALDI, an AB SCIEX TOF/TOF 5800 and a Waters Synapt G2. AuNPs also offer a straight-forward platform for functionalization using gold-thiol chemistry. Here we used two separate commercially available thiols, 1H,1H,2H,2H-perfluorodecanethiol (fC10) and 1H,1H,2H,2H-perfluorooctanethiol (fC8). However, there is also the opportunity to design new ligands for the AuNPs that could enhance ionization, for example, amine fluorocarbon ligands could facilitate desorption/ionization of negatively charged metabolites since the ligand’s amine would act as a proton acceptor. Soft ionization with fluorinated AuNPs To illustrate the laser-induced thermal energy generated at f-AuNPs, 4-nm f-AuNPs were measured with transmission electron microscopy (TEM) before and after laser irradiation ( Fig. 2 ). The size distribution in the top panel of Fig. 2 shows an increase in size (to ~6 nm) indicating that the particles melt and anneal following exposure to the laser pulses. The accompanying TEM images in Fig. 2b offer further evidence that laser radiation has melted and fused the f-AuNPs. The thermal energy responsible for melting the particles can be used to desorb the fluorocarbon ligand, thus indirectly desorbing analyte molecules into the gas phase for mass spectrometry analysis. Thermal desorption, however, typically requires high energy, which leads to significant fragmentation, including the formation of ions that are primarily cation adducts [33] and the formation of gold cluster ions [37] . Therefore, our next set of experiments explored the performance of the f-AuNPs and whether thermal release of the fluorocarbon ligand was beneficial to the mass spectrometry analyses. To do this, the f-AuNPs were compared with MALDI and AuNPs functionalized with the non-fluorous ligand octanethiol (C8-AuNPs) by tracking the survival yield of the thermally labile molecule methoxybenzyl pyridinium with respect to laser energy ( Fig. 2 ). Survival yield was calculated as the ratio of [M] + ( m/z =200) to the major fragment at m / z =121. Desorption of methoxybenzyl pyridinium was initiated at energies above 0.78 μJ; when using MALDI with α-cyano-4-hydroxycinnamic acid, (C8-AuNP) initiated desorption at energies above 0.50 μJ, while the f-AuNP initiated desorption at energies above 0.25 μJ for the 8-carbon fluorous ligand (F8-AuNP) and 0.34 μJ for the 10-carbon fluorous ligand (F10-AuNP). The low-energy behaviour of f-AuNPs allows NIMS experiments to be carried out at energies that are below the threshold for gold cluster formation ( Supplementary Fig. 3 ), a significant advantage since these ion clusters can complicate the mass spectrum in the low mass region. In addition, the low energies used tend to create minimal background signal compared with typical MALDI matrices ( Supplementary Figs 4–15 ). 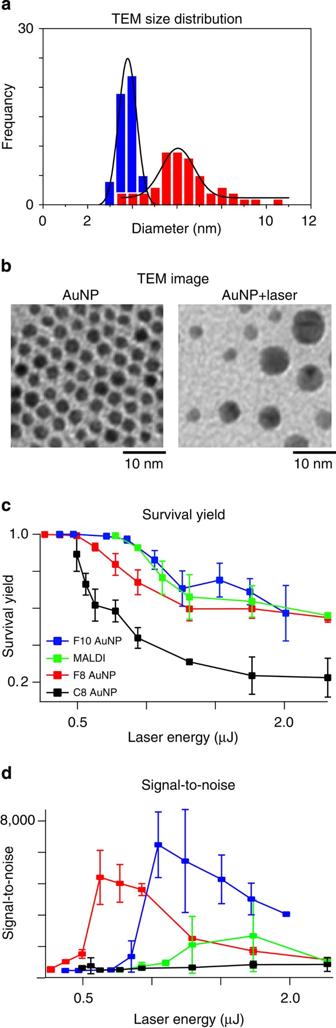Figure 2: Soft ionization with f-AuNPs. (a) The diameter of AuNPs increases from 3.5±0.5 nm to 6.0±1.4 nm after laser irradiation. (b) TEM images of AuNPs before and after laser irradiation. Scale bar, 10 nm. (c) Survival yield versus laser energy plot of methoxybenzyl pyridinium for F8-AuNP, F10-AuNP, C8-AuNP and MALDI (error bars are s.d.). (d) Signal-to-noise versus laser energy plot for [M]+(m/z=200) for F8-AuNP, F10-AuNP, C8-AuNP and MALDI (error bars are s.d.). Figure 2: Soft ionization with f-AuNPs. ( a ) The diameter of AuNPs increases from 3.5±0.5 nm to 6.0±1.4 nm after laser irradiation. ( b ) TEM images of AuNPs before and after laser irradiation. Scale bar, 10 nm. ( c ) Survival yield versus laser energy plot of methoxybenzyl pyridinium for F8-AuNP, F10-AuNP, C8-AuNP and MALDI (error bars are s.d.). ( d ) Signal-to-noise versus laser energy plot for [M] + ( m/z =200) for F8-AuNP, F10-AuNP, C8-AuNP and MALDI (error bars are s.d.). Full size image The survival yield plot in Fig. 2 shows that the f-AuNPs performed exceptionally well in terms of fragmentation as compared with the C8-AuNPs. We observed that fragmentation begins immediately at the threshold energy required for desorption and levels out at ~20% survival for C8-AuNP, whereas the F8-AuNP maintained 100% survival over 0.25–0.50 μJ and reached a steady state of 60% at 1.25 μJ. These results suggest that the fluorous-thiol functionality effectively insulates the sample from the potentially damaging thermal energy from the irradiated AuNPs. This is further evidenced by the observation that the longer fluorinated alkane thiol functionalized F10-AuNPs maintain 100% survival over a longer range (0.34–0.80 μJ) as presumably the longer chain better insulates the analyte from the heat generated at the particle surface. It is also interesting to note that fragmentation begins at energies far below the threshold for desorption of bare nanoparticles, showing the inherent harshness of nanoparticle-based thermal desorption. The comparison to be made with MALDI-MS is more nuanced; at very low energies, desorption does not occur in MALDI-MS, while it does occur using f-AuNP with essentially no damage to the molecular ion. As the energy approaches the threshold for MALDI, the survival yield for f-AuNPs begins to decrease and continues to decrease at a slower rate than MALDI until both desorption methods reach a steady state of 60% at 1.25 μJ. Generally, we observed that the f-AuNPs outperform MALDI at low energy and perform comparably at higher energies. The signal-to-noise ratios plotted in Fig. 2 show that the particles perform better than both MALDI and the C8-AuNP in terms of the generation of [M] + signal. This result is again most likely due to the low energy requirements for this type of desorption/ionization. In addition, the longer chain appears to perform slightly better than the shorter chain. The length of the chain appears to shift and extend the optimal energy range for this experiment; however, in both cases, it should be noted that the maximum signal-to-noise occurs at energies above 100% survival. Furthermore, it could be the case that the trend would continue with the use of a perfluorododecanethiol (F12); however, this ligand was not readily available. In addition to the low-energy requirements of the f-AuNP observed in the survival yield experiments, scanning electron microscopy (SEM) data indicate that the desorption process is particularly soft. Unlike the typical ablation ‘craters’ observed in MALDI-MS analysis of the tissue ( Supplementary Fig. 16 ), we observed plateau-like structures in the f-AuNP experiments. 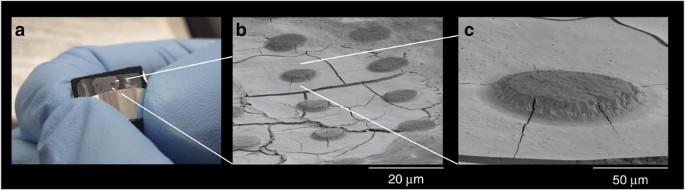Figure 3: Characterization of desorption/ionization using fluorinated nanoparticles. (a) Silicon substrate with a thaw-mounted section of mouse lung spotted with a f-AuNP solution. (b) SEM characterization of the mouse lung section spotted with f-AuNPs after laser irradiation. (c) The plateau-shaped spots (50–60 μm in diameters) formed on the tissue surface after laser irradiation. Figure 3 shows a slice of lung tissue that was spotted with the f-AuNP solution and irradiated with a Nd:YAG laser. In the treated area, the laser pulses create raised protrusions. Outside of this f-AuNP-coated region, no protrusions were formed. Interestingly, the laser pulses that occurred at the interface create partial plateau structures. We suspect that the protrusion of the surface following laser radiation is a side product brought about by the heating of the f-AuNPs. We speculate that the heat of the f-AuNPs vaporizes the more volatile components in the tissue, creating the plateau-like effect, however this phenomenon requires further investigation. Figure 3: Characterization of desorption/ionization using fluorinated nanoparticles. ( a ) Silicon substrate with a thaw-mounted section of mouse lung spotted with a f-AuNP solution. ( b ) SEM characterization of the mouse lung section spotted with f-AuNPs after laser irradiation. ( c ) The plateau-shaped spots (50–60 μm in diameters) formed on the tissue surface after laser irradiation. Full size image NIMS and SEM imaging of biofilms The overarching goals of this technology are to increase both the accessibility and the functionality of nanostructure-based imaging. Using f-AuNPs as a platform accomplishes these goals by adding multiple methods of imaging capabilities. To this point, another advantage of f-AuNPs is their solubility in biologically inert fluorocarbon solvents that can be applied to the top of a tissue sample. This contrasts to classic silicon NIMS experiments, which require that the sample be thinly sliced and placed on top of a nanostructured surface. We tested the versatility of the f-AuNPs on a biofilm sample that would not be immediately accessible to silicon nanostructure-based techniques due to the thickness of the sample [38] . To analyse these samples, the aclar substrates that the biofilms were grown on were attached directly to the target plate where, following desiccation, the f-AuNPs were deposited drop wise. The NIMS data shown in Fig. 4 illustrate that f-AuNP can be used to initiate desorption/ionization from these irregular biofilm surfaces. This image compares two biofilm cultures of Desulfovibrio vulgaris (DVH)—one that was grown in balanced conditions and one that was grown in stressed conditions. Stressed conditions refer to an electron acceptor-limited (EAL) environment, which affects the biofilm growth of sulfate reducing bacteria, like DVH. The mass spectra extracted from the balanced and stressed bacteria ( Fig. 4 ) show several differences, the most dramatic one at m / z 551, which has been mapped to the right of the mass spectra in Fig. 4 . This ion was putatively identified ( Supplementary Fig. 17 and Supplementary Table 1 ) diglyceride (16:0/16:0) (ref. 39 ) and might be indicative of perturbed metabolism in the stressed bacteria; however, this is still a very preliminary finding. In addition, f-AuNPs were successfully applied to the bacteria sample, following fixation and dehydration, to act as a contrast agent for the comparatively high-resolution SEM images shown in Fig. 4 . Surprisingly, we found that the density of the EAL bacteria was in fact increased relative to the balanced bacteria. This result was confirmed using a standard SEM procedure and is currently under further investigation. 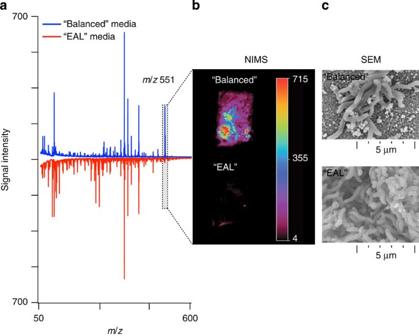Figure 4: NIMS and SEM imaging using fluorinated AuNPs. (a) Mass spectra generated from two regions of interest in the f-AuNP MSI—one corresponds to the biofilm grown in balanced media (blue) and one corresponding to the biofilm grown in EAL media (red). The inset (b) shows the ion image form/z551. (c) SEM images of balanced and stressed biofilms treated with f-AuNP. Figure 4: NIMS and SEM imaging using fluorinated AuNPs. ( a ) Mass spectra generated from two regions of interest in the f-AuNP MSI—one corresponds to the biofilm grown in balanced media (blue) and one corresponding to the biofilm grown in EAL media (red). The inset ( b ) shows the ion image for m / z 551. ( c ) SEM images of balanced and stressed biofilms treated with f-AuNP. Full size image NIMS and X-ray μCT imaging of mouse lung tissue The success of the mass spectrometric detection of metabolites using f-AuNPs ( Fig. 4 ) has allowed for the further integration of the f-AuNPs NIMS analysis with μCT. Together these two modes of imaging allow for the correlation of three-dimensional anatomical (structural) and molecular information ( Supplementary Fig. 18 ). For example, this has been demonstrated in the analysis of metastatic mouse lungs. Specifically, 500 μl of the biologically inert f-AuNP solution was intratracheally introduced into mouse lungs and immediately distributed into the lung tissue. The liquid ventilated lung was then embedded into OCT (optimal cutting temperature) material and preserved in −80 °C until analysis. The mouse lung was then imaged with μCT to construct high-resolution three-dimensional image ( Fig. 5 Supplementary Video 1 ). F-AuNPs were well distributed into the lung tissue and characterized the airway and porosity of the lung. The blood vessels appear as dark areas and the regions of the lungs carrying metastases revealed dark spots consistent with the exclusion of nanoparticle from the metastatic lesions ( Supplementary Fig. 19 ). 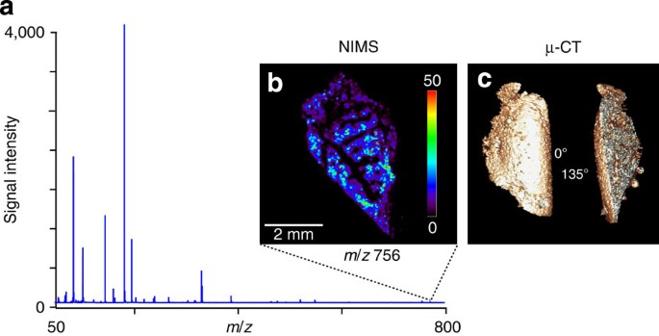Figure 5: NIMS and μCT imaging using fluorinated AuNPs. (a) Mass spectra generated from a single-lobe metastatic mouse lung ventilated with f-AuNPs. The inset (b) shows the ion image form/z756. (c) μCT images of the same lobe of the f-AuNP-ventilated metastatic mouse lung at 0° and 135° where gold indicates the surfaces of the f-AuNP-ventilated lung and silver represents the volume. Figure 5: NIMS and μCT imaging using fluorinated AuNPs. ( a ) Mass spectra generated from a single-lobe metastatic mouse lung ventilated with f-AuNPs. The inset ( b ) shows the ion image for m / z 756. ( c ) μCT images of the same lobe of the f-AuNP-ventilated metastatic mouse lung at 0° and 135° where gold indicates the surfaces of the f-AuNP-ventilated lung and silver represents the volume. Full size image To obtain molecular information from liquid ventilated metastatic lung tissue, OCT-embedded lungs were sectioned (20 μm) and analysed. Since the f-AuNPs solution had been passed through the trachea into the lung, no additional f-AuNPs were applied to the tissue. A mass spectrometry image of the f-AuNP-ventilated left lobe of the lung is shown in Fig. 5 . In general, mass spectrometry analysis is a multiplexed analysis where multiple molecular ions can be simultaneously detected in one experiment. Here we chose to map a phosphatidylcholine ( Supplementary Fig. 20 ) at m / z 756 to demonstrate molecular information and its distribution in this tissue ( Fig. 5 ). To confirm that the areas lacking nanoparticle signal did contain cancerous tissue, metastases in an intact liquid ventilated mouse lung were identified by haematoxylin and eosin staining and compared with an adjacent NIMS image ( Supplementary Fig. 19 ). To better access these structures, it might be possible to approach the metastases from the blood stream by perfusing the animal with a synthetic blood form of the f-AuNP or to coat the tissue following sectioning ( Supplementary Fig. 21 ). To enable NIMS and X-ray μCT imaging of blood vessels in situ , we took advantage of fluorocarbons utility as a blood substitute [2] , [40] . The f-AuNPs were dissolved in the fluorocarbon perfluordecalin, which was emulsified to approximate the only the Food and Drug Administration-approved fluorocarbon-based blood substitute [40] . The f-AuNP emulsion was perfused into the circulatory system to demonstrate the ability to obtain structural and chemical information from the circulatory system associated with the lung ( Supplementary Fig. 22 ) as well the liver ( Supplementary Fig. 23 ) of the mouse. In addition, we also applied these imaging approaches to investigate the structural and chemical effects of hyperoxia on the lung tissue of juvenile mice ( Supplementary Figs 24 and 25 ). NIMS for analysis of central carbon metabolites The majority of central carbon metabolites are anionic and thus are better suited for analysis in negative ion mode imaging mass spectrometry. One successful approach used for the in situ ionization and imaging of central carbon metabolites employs amine-functionalized initiators [30] and MALDI matrices [31] . Presumably, these adjuvants work well because the basic amine group acts as a proton acceptor to promote M−H − production. Thus, to enable the application of this imaging platform to the analysis of central carbon metabolites in negative ionization mode, we have to enrich the fluorocarbon solvent with the basic initiator 1H,1H,2H,2H,3H,3H-perfluoroundecylamine (PFUA). As it was not clear that the f-AuNPs would transfer the requisite energy to the initiator molecule needed to induce desorption/ionization, we tested the enriched f-AuNPs using a standard mixture of nine metabolites in negative mode. A mass spectrum generated from this experiment is shown in Fig. 6 ; in addition to the peaks for each individual metabolite, we also observe peaks for Au − and PO 4 H 2 − . We attribute the emergence of these ions to the higher energy used in this experiment. The spectra in Supplementary Fig. 3 show that under the standard operation energy of 1.4 μJ no Au ions are formed; the addition of PFUA, however, increased the energy requirement to ~2 μJ. Just as the energy threshold increases with chain length ( Fig. 2 ), the incorporation of the PFUA shifted this threshold even further by ostensibly adding a second barrier between the AuNP and the analyte. However, even at this increased energy, the enriched f-AuNPs performed well in negative ion mode. 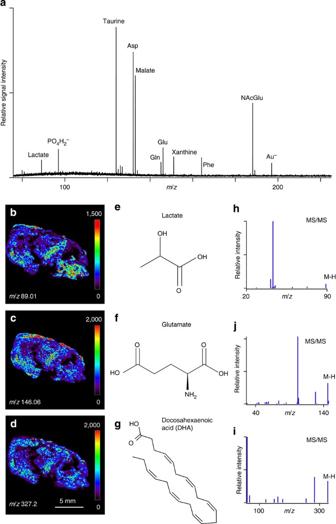Figure 6: NIMS for the analysis of central carbon metabolites. (a) A mass spectrum for nine metabolites in a standard mixture. (b–d) NIMS images of a sagittal slice of a mouse brain collected in negative ion mode. Each image is paired with (e–g) the structure of the identified metabolite and (h–j) tandem MS data that were collected using LC-MS/MS. Figure 6: NIMS for the analysis of central carbon metabolites. ( a ) A mass spectrum for nine metabolites in a standard mixture. ( b – d ) NIMS images of a sagittal slice of a mouse brain collected in negative ion mode. Each image is paired with ( e – g ) the structure of the identified metabolite and ( h – j ) tandem MS data that were collected using LC-MS/MS. Full size image The enriched f-AuNPs were then used to demonstrate central carbon metabolite imaging in tissue using negative ionization mode. The enriched particles were applied to the top of a sagittal slice from one half of a bifurcated mouse brain after desiccation. In Fig. 6 , we have mapped the ions corresponding to lactate, glutamate and docosahexenoic acid. The presence of each mapped metabolite was then confirmed by LC-MS/MS analysis of the second half of the brain. Here we have demonstrated that this platform like Si-based NIMS [30] has the ability to use specialized initiators to expand the number of metabolites that are amicable to mass spectrometry imaging. Fluorinated AuNPs (f-AuNPs) were designed to facilitate NIMS as well as act as contrast agents for EM and μCT. An important feature of the f-AuNPs is that they promote a gentle laser desorption/ionization mechanism facilitating intact molecular ion formation with little background interference or molecular ion fragmentation. The utility of AuNPs for structural μCT measurements is well established but the primary advance of employing fluorinated ligands to these structures has allowed for structural data (μCT) to be combined for the first time with molecular mass spectrometry information (f-AuNPs NIMS). This multimodal imaging approach is particularly useful for performing mass spectrometry-based metabolite imaging, where correlating metabolite concentrations with anatomical structure is key to data interpretation. The fluorocarbon liquid component of the method affords versatility in the delivery of the agent, which can be carried out via direct coating, liquid ventilation or perfusion allowing analysis of morphologically diverse biological samples. Chemicals Octanethiol-functionalized AuNPs (2–4 nm DLS, 2% w/v in toluene) and fluorinated ligands 1H,1H,2H,2H-perfluorodecanethiol (fC10) and 1H,1H,2H,2H-perfluorooctanethiol (fC8), methoxybenzyl pyridinium chloride and perfluorodecalin were purchased from Sigma-Aldrich (St Louis, MO, USA) and 10% Gibco Pluronic F-68 was from Life Technologies (Grand Island, NY) 1H,1H,2H,2H,3H,3H-perfluoroundecylamine was from Santa Cruz Biotechnology (Dallas, TX). Nanoparticle synthesis Octanethiol-functionalized AuNPs were in toluene with a concentration of 20 mg ml −1 . One ml of octanethiol-functionalized AuNPs (20 mg) was added to ~20 ml of ethanol to precipitate the AuNPs with centrifugation at 4,000 r.p.m. for 15 min. The precipitated AuNP were then washed with acetone, briefly sonicated and centrifuged again. The cleaning procedure was repeated three times before being dissolved in 1 ml of hexane. The AuNP solution (1 μl) was then analysed using LDI-MS to test for the presence of tetraoctyl ammonium bromide by monitoring the tetraoctyl ammonium ion at m/z 466, which is commonly used as a phase transfer additive in nanoparticle synthesis. More acetone washes were conducted until tetraoctyl ammonium ion was not detected. An additional 1 ml of hexane and 400 μl of 1H,1H,2H,2H-perfluorooctanethiol (fC8) or 1H,1H,2H,2H-perfluorodecanethiol (fC10) was added and the vial was purged with nitrogen gas to remove air. The solution was stirred for one to three days until AuNPs precipitated. The solvent was evaporated with nitrogen gas flow and nanoparticles were washed three times with hexane, three times with acetone and two times with 1:1:1 methanol/acetone/water, respectively, to remove excess ligand and impurities. Following washing, the AuNP was dried in the oven (~80 °C) for several minutes and stored as a solid. Before use, the AuNP was dissolved in tetradecafluorohexane (PFH) at 3 mg ml −1 for mass spectrometry and electron microscopy analyses and 10 mg ml −1 in perfluorodecalin for mouse lung perfusion experiments. Enriched f-AuNPs were made by dissolving 3 mg ml −1 f-AuNPs into 5% 1H,1H,2H,2H,3H,3H-perfluoroundecylamine perfluorodecalin solution. The blood substitute f-AuNP solution was made by combining 50% 20 mg ml −1 f-AuNP/prefluorodecilin and 50% Pluronic F-68 (0.5%) in Milli-Q water. The immiscible solutions were sonicated for 5 min at 50% duty cycle with a probe sonicator. Electron microscopy characterization For TEM imaging, fluorinated AuNPs were deposited on 400 mesh copper grids and characterized by a Philips CM100 electron microscope (FEI, Hillsborough, OR) at 80 kV. Images were collected using a Megaview III CCD camera (Olympus Soft Imaging Solutions, Münster, Germany). Fluorinated AuNPs deposited on copper grids were also irradiated with (355 nm, laser energy 6.6 μJ, 2,000 shots), and then measured with TEM. For SEM analysis, 10 μl of 3 mg ml −1 fluorinated AuNPs in PFH were first deposited onto mouse brain or lung tissue which was then irradiated by a laser with a predefined 250-μm step size. Subsequently, the samples were imaged with a Hitachi S4800 SEM at 5 kV. SEM was done on biofilms from the same batch. Aclar slides with adhered biofilm were aldehyde fixed (2.5% w/v glutaraldehyde, 2.0% w/v paraformaldehyde, 0.05 M sodium cacodylate buffer pH 7.0) overnight. Samples were rinsed with double-distilled H 2 O and ethanol dehydrated. Critical point drying was then carried on the samples using CO 2 and spotted with f-AuNP solution (1 mg ml −1 ). Samples were also viewed on a Hitachi S4800 SEM. Bacterial strains and growth conditions DVH RCH1 was obtained from Dr Romy Chakraborty (Lawrence Berkeley National Lab) and was isolated from Cr-contaminated groundwater at the U.S. Department of Energy Hanford reservation. DVH RCH1 was grown in LS4D medium, which contains lactate as the carbon source and electron donor and sulfate as the electron acceptor [41] . Lactate and sulfate concentrations were altered to create balanced and EAL conditions. The balanced condition was defined as 60 mM sodium lactate and 30 mM sodium sulfate and the EAL condition was defined as 50 mM sodium lactate and 10 mM sodium sulfate. DVH RCH1 was grown as a biofilm under continuous flow conditions in a modified Center for Disease Control reactor. Exponential phase cells were inoculated into a reactor containing balanced or EAL lactate–sulfate media (LS4D) and were grown in batch mode for 48 h. Biofilms were grown at room temperature (20–23 °C), with a dilution rate of 0.04 per hour, stirred at 60 r.p.m. and the headspace was continually purged with sterile N 2 gas to maintain anaerobic conditions. Coupons of aclar (7.8 m.i.l. thickness; Electron Microscopy Sciences, Hatfield, PA) supported by glass slides were submerged in the reactor body as a surface for biofilm growth. Aclar coupons were removed from the reactor after 144, rinsed three times in ice-cold PBS, wicked dry and flash frozen in liquid nitrogen. Samples were stored at −80 °C until analysis. Animals and μCT imaging All animal work complied with the National Institutes of Health and institutional guidelines (TSRI is AAALAC, International accredited). Female 11-week-old CB17- Prkdc SCID mice were euthanized by overdose of isoflurane before exsanguination by cutting the abdominal aorta. A small incision was performed in the trachea to insert a 20 gauge blunt needle, which was secured by a piece of suture. Approximately 500 μl of 10 mg ml −1 f-AuNP in PFH solution was then injected into the lungs up to full lung inflation. Intact lungs were immediately harvested, placed in OCT compound embedding medium, frozen in liquid nitrogen and stored at −80 °C before analysis. For the hyperoxia experiment, the experimental group consisted of C57BL/6J P7 pups (7 days old) exposed to 75% oxygen for 5 days and returned to room air at P12 (12-day-old pups). The control group consisted of age-matched pups raised in normoxia (21% O2) for the same period. Pups were killed at P12. As was the case with adult mice, the pups were euthanized by overdose of isoflurane before exsanguination by cutting the abdominal aorta. Ventilation of the f-AuNPs in this case was carried out directly via the mouth to the trachea. Approximately 250 μl of 10 mg ml −1 f-AuNP in perfluorodecalin solution was then injected into the lungs up to full lung inflation. Again, the intact lungs were immediately harvested, placed in OCT compound embedding medium, frozen in liquid nitrogen and stored at −80 °C before analysis. For the blood substitute experiment, a male mouse (C57BL/6J, 24 days of age) was anaesthetized with isoflurane and the heart was exposed. A 23-gauge needle attached by tubing to a syringe was inserted into the left ventricle, the right atria was pierced and 40 ml saline was perfused through the animal at a rate of 3.1 ml min −1 to clear all of the blood. A three-way valve was switched so that 3 ml of the f-AuNP blood substitute was then pumped through the mouse at the same rate. The lung and liver were harvested and imbedded in OCT until μCT analysis. The intact mouse lungs and liver were imaged by μCT (vivaCT 75; Scanco Medical AG; Basserdorf, Switzerland) in standard resolution using the following parameters: 55 kVP, 145 μA, 300-ms integration time and 41-μm voxel size. The scanning protocol was programmed to acquire images via a rotating gantry, resulting in a total of 500 step-projections per scan. The projections were reconstructed with a matrix of 1,024 × 1,024 using Scanco’s μCT Tomography V5.4C software. The two-dimensional binary digital imaging communication files obtained from Scanco’s software were later analysed using 64-bit OsiriX v.3.9.2 (Pixmeo; Geneva, Switzerland) software. Mass spectrometry analysis and imaging For the analysis of standard compounds, 0.5 μl of f-AuNP solution (3 mg ml −1 ) was first deposited onto a p -type silicon chip and allowed to air dry. Then, 0.1–0.5 μl of standard compound solution was deposited on top of dried f-AuNP layer and dried under vacuum. An AB SCIEX TOF/TOF 5800 MS system was used for data collection. The instrument was operated at reflectron mode with a repetition frequency of 400 Hz and an accelerating voltage of 15 kV. Each sample spectrum was averaged from 400 laser shots. Plasma was analysed using a MALDI SYNAPT G2S (Waters, Milford, MA) equipped with a Nd:YAG laser (355 nm) with a repetition frequency of 1,000 Hz and variable laser energy (8–10 μJ). Nitrogen was used in the ion mobility cell and the mobility experiments were collected with a variable wave velocity of 320 to 900 m s −1 for the 50 to 1,200 m / z region. Mouse lung and liver tissue treated with AuNPs was sliced with a Leica CM1900 cryostat to a thickness of 20 μm, and then thaw-mounted directly onto p -type silicon chip. The tissues were directly imaged by an AB SCIEX TOF/TOF 5800 MS system without additional sample preparation. Tissue slices were imaged with a 100 μm step size and each recorded mass spectrum resulted from the average of 400 laser shots. Representative sections of the cancer metastasized lungs were collected on Superfrost Plus slides and stained with hematoxylin and eosin using routine histological techniques. LC-MS/MS Lung tissue and biofilm samples were analysed using reversed phase liquid chromatography/MS analysis in ESI-positive mode. The extracts were analysed on 6550 iFunnel QTOF mass spectrometer (Agilent Technologies) interfaced with 1200 series HPLC system (Agilent Technologies). For reversed phase liquid chromatography separation, 0.1% formic acid in water was used as mobile phase A and 0.1% formic acid in acetonitrile was used as mobile phase B. The metabolite extract was loaded onto a C18 column using 5% mobile phase B at a flow rate of 100 μl min −1 and resolved using a linear gradient of 5% B–95% B over 60 min. How to cite this article : Kurczy, M. E. et al . Comprehensive bioimaging with fluorinated nanoparticles using breathable liquids. Nat. Commun. 6:5998 doi: 10.1038/ncomms6998 (2015).